The critical size is set at a single-cell level by growth rate to attain homeostasis and adaptation Budding yeast cells are assumed to trigger Start and enter the cell cycle only after they attain a critical size set by external conditions. However, arguing against deterministic models of cell size control, cell volume at Start displays great individual variability even under constant conditions. Here we show that cell size at Start is robustly set at a single-cell level by the volume growth rate in G1, which explains the observed variability. We find that this growth-rate-dependent sizer is intimately hardwired into the Start network and the Ydj1 chaperone is key for setting cell size as a function of the individual growth rate. Mathematical modelling and experimental data indicate that a growth-rate-dependent sizer is sufficient to ensure size homeostasis and, as a remarkable advantage over a rigid sizer mechanism, it reduces noise in G1 length and provides an immediate solution for size adaptation to external conditions at a population level. Cell size can be considered as the outcome of complex parallel and interconnected processes that convey different sorts of intrinsic and extrinsic information. Of all these processes, cell growth and cell cycle are particularly relevant as they likely apply to all organisms, and their efficient and precise coordination is a fundamental biological problem [1] , [2] , [3] , [4] , [5] , [6] , [7] , [8] , [9] , [10] . As a unicellular eukaryote, Saccharomyces cerevisiae has been widely used to study the mechanisms that determine cell size, mainly because this budding yeast displays two of the most universal properties regarding cell size control, a constant mass/ploidy ratio [11] and a critical size threshold for cell cycle progression [12] , [13] , which is mainly exerted at Start, a key event in late G1. Two heteromeric transcription factors [14] , SBF (Swi6–Swi4) and MBF (Mbp1–Swi6), drive a transcriptional wave of ~200 genes [15] at Start to initiate budding and trigger S-phase entry. The most upstream activator of Start is a complex formed by Cln3 [16] , [17] , [18] , [19] , [20] , a G1 cyclin, and Cdc28 [21] , the cyclin-dependent kinase that controls the cell cycle in budding yeast. The Cdc28–Cln3 complex phosphorylates Whi5 (and presumably Swi6) at multiple residues to activate SBF- and MBF-dependent transcription [22] , [23] in a scheme homologous to the onset of the mammalian cell cycle, where Cdk4,6–cyclin D complexes phosphorylate retinoblastoma protein (pRB) to activate E2F–DP transcription factors [24] . Two other G1 cyclins, Cln1 and Cln2, are upregulated by SBF and have a key role with Cdc28 in a positive feedback loop essential for coherent and irreversible execution of Start [25] , [26] , [27] . The Cln3 cyclin is present at constant levels throughout G1 [19] , [28] and it is regulated by a retention/release mechanism that prevents its unscheduled accumulation in the nucleus [29] . Whi3, first identified as a negative regulator of Cln3 activity [30] , binds the CLN3 mRNA and recruits Cdc28 to help retain newly formed Cdc28–Cln3 complexes at the endoplasmic reticulum (ER) during early and mid G1 [31] , [32] , [33] . In late G1, the Ydj1 chaperone has an essential role in releasing Cln3 or the Cdc28–Cln3 complex from the ER [33] , which allows its accumulation in the nucleus to phosphorylate Whi5 and trigger Start. Screens for small-cell-size mutants have not only identified key proteins of the Start network, such as Cln3, Whi3 and Whi5, but also central regulators of ribosome biogenesis [34] , namely Sfp1 and Sch9, indicating a close functional interaction between the machineries that control growth and proliferation [4] . On the other hand, and in addition to its role at Start, Ydj1 is heavily involved in protein translocation across the ER membrane [35] , a key process for cell growth. These lines of evidence suggest that the critical size could be set by mechanisms intimately linked to cell growth [4] , [29] . Although it is generally accepted that budding yeast cells must grow to reach a critical size before cell cycle entry [4] , [10] , [12] , [13] , cell volume at Start displays a very large variability under constant conditions [36] , which strongly argues against the existence of a deterministic mode of cell size control. This key question has been analysed recently at a single-cell level, and it was proposed that cell size variability at Start is mainly due to molecular noise intrinsic to the mechanisms that activate the G1/S regulon [37] . Here we show that most of the large variation in cell size at Start is not because of an inherent stochastic behaviour. Instead, cell size at Start is an individual parameter robustly set by the rate at which each individual cell grows during G1. We also show that the growth-rate-dependent sizer is intimately hardwired into the Start network, the Ydj1 chaperone being the most important factor for setting the critical size as a function of the individual growth potential. We also show that a growth-rate-dependent sizer ensures size homeostasis and gives a simple solution to cell size adaptation to different external conditions as long as they have an impact on growth rate. Moreover, as a notable advantage over the constant critical size postulated up to now, a growth-rate-dependent sizer reduces noise in G1 length and equalizes the generation time of fast- and slow-growing cells, thus maintaining cell diversity at a population level. Discontinuous growth and cell-to-cell variability As a first step to investigate interdependencies between growth and cell cycle entry at a single-cell level, we first determined volume growth kinetics of newborn cells by time-lapse microscopy ( Fig. 1a , Supplementary Movie 1 ). Accurate volumetric data were obtained by means of a densitometric profile along radial axes to iteratively detect the optical boundary of the cell ( Fig. 1b , Supplementary Movie 2 ) and obtain its volume assuming a prolate spheroid as shape. Volume distributions and average growth rates obtained by time-lapse microscopy were similar to those obtained with a Coulter Counter in batch cultures ( Supplementary Fig. S1 ). Using this methodological approach, we observed a clearly discontinuous pattern of growth in volume during the cell cycle ( Fig. 1c ). First, cell volume increased in a fairly constant manner throughout G1, with only a slight decrease in the rate immediately before budding. Of particular relevance to the hypothesis of this work (see below), we observed a large cell-to-cell variability in volume growth rate during G1 similar to that observed in other biosynthetic processes [38] , [39] , [40] ( Supplementary Fig. S2 ). On the other hand, a strong increase in volume growth rate was observed approximately 20 min after budding, which decreased again to initial values by the end of the cell cycle ( Fig. 1d, e ). Thus, average volume growth rate in G2–M increased 2.3-fold compared with G1 phase, but individual rates in the two periods were not correlated significantly ( Supplementary Fig. S2 ). This pattern of growth in volume was very similar in a different strain background ( Supplementary Fig. S3 ). Overall, our data support previous studies that have proposed a rate-change point (RCP) for growth in volume shortly after budding [41] , [42] . 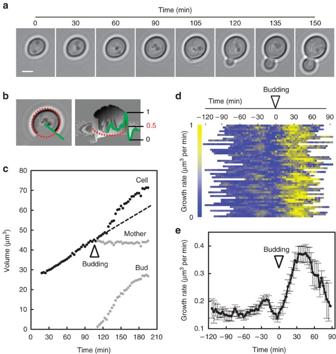Figure 1: Volume growth during the cell cycle of budding yeast. (a) Time-lapse microscopy images of an elutriated daughter cell during entry into the cell cycle in SC plus glucose. Bar=2 μm. (b) Accurate determination of cell volume from bright-field images. A radial density profile (green line) was used to find two consecutive maximum and minimum pixel values across the cell boundary, which was then arbitrarily established at a pixel which has the value of their arithmetic greyscale mean (seeMethodsfor details). Cell boundary pixels (red dots) were iteratively defined by a full rotation of the radial axis, an ellipse was fitted to the resulting polygon, and major and minor axes were finally used to calculate the cell volume assuming a prolate as shape. (c) Time-lapse images from cell shown inawere used to determine volume growth kinetics during a full cell cycle. Bud and mother cell compartments were separately analysed after budding. (d) Heat map generated from instantaneous growth rates in volume during the cell cycle of elutriated daughter cells (n=50). Instantaneous rate values were obtained as described under Methods and aligned at budding time (t=0) for each cell. (e) Mean values of instantaneous growth rates in volume during in G1 from cells indand corresponding confidence limits (significance level of 0.05) are plotted. Figure 1: Volume growth during the cell cycle of budding yeast. ( a ) Time-lapse microscopy images of an elutriated daughter cell during entry into the cell cycle in SC plus glucose. Bar=2 μm. ( b ) Accurate determination of cell volume from bright-field images. A radial density profile (green line) was used to find two consecutive maximum and minimum pixel values across the cell boundary, which was then arbitrarily established at a pixel which has the value of their arithmetic greyscale mean (see Methods for details). Cell boundary pixels (red dots) were iteratively defined by a full rotation of the radial axis, an ellipse was fitted to the resulting polygon, and major and minor axes were finally used to calculate the cell volume assuming a prolate as shape. ( c ) Time-lapse images from cell shown in a were used to determine volume growth kinetics during a full cell cycle. Bud and mother cell compartments were separately analysed after budding. ( d ) Heat map generated from instantaneous growth rates in volume during the cell cycle of elutriated daughter cells ( n =50). Instantaneous rate values were obtained as described under Methods and aligned at budding time ( t =0) for each cell. ( e ) Mean values of instantaneous growth rates in volume during in G1 from cells in d and corresponding confidence limits (significance level of 0.05) are plotted. Full size image Cell size at Start is dictated by volume growth rate in G1 We next extended our analysis to determine cell volume at Start, when nuclear export of the transcriptional repressor Whi5 takes place [23] , [43] . Elutriated and asynchronously growing daughter cells were analysed using time-lapse microscopy ( Supplementary Movies 3 and 4 , respectively), and a Whi5—green fluorescent protein (GFP) nuclear index was quantified to determine cell volume at Start ( V s), time at Start ( T 1) and volume growth rate in G1 ( α ; Fig. 2a,b ; Supplementary Fig. S4 ). Although we assumed linear kinetics to obtain volume growth rates in G1 as the simplest approximation to our data ( Fig. 1c–e ), very similar results were obtained if exponential kinetics were assumed (data not shown). Although there was no correlation between volume and time at Start, volume at Start was closely correlated with volume growth rate in G1 ( Fig. 2c,e ; Supplementary Tables S1 and S2 ), giving support to the hypothesis that individual growth rate could be a key determinant of cell size at Start [4] , [29] . If G1 length were a constant, this finding could have an obvious explanation, but this is not the case. First, time at Start fluctuated over a tenfold range, whereas volume at Start only varied across a threefold range. Second, time at Start did not correlate with growth rate ( Fig. 2g ; Supplementary Table S3 ). Finally, relative s.e. for volume and time at Start estimated from growth rate were 7.5% and 44.7%, respectively, which makes time a very unlikely determinant of volume at Start as a function of growth rate. As nutrients are potent modulators of growth rate in yeast, we analysed cells growing asynchronously in different carbon sources, and we found that volume at Start correlated with volume growth rate in G1 not only for each nutritional condition considered separately, but also when all results were pooled ( Fig. 2d ; Supplementary Table S1 ). As discussed above, it is very unlikely that time at Start mediates this correlation ( Fig. 2h ). Time from Start to budding ( T 2) showed less variability [43] and it did not correlate with growth rate ( Supplementary Fig. S5 ). Overall, our data suggest that individual growth rate determines cell volume at Start independently of the nutritional environment. 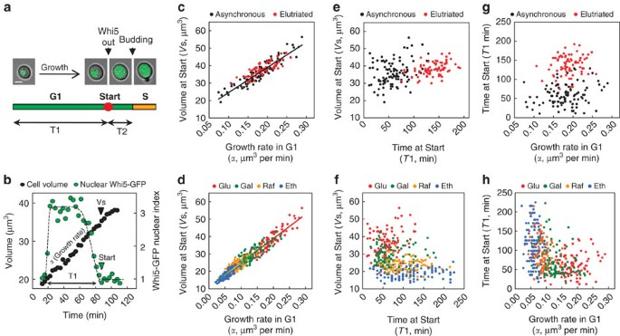Figure 2: Volume at Start correlates with volume growth rate in G1 at a single-cell level. (a) Start can be defined as the event where Whi5 is exported from the nucleus23,43. Thus, time at Start (T1) was determined as the period where Whi5 was nuclear, whereas time to budding (T2) was the period from Whi5 exit from the nucleus to budding. Bar=2 μm. (b) Cell volume (black circles) and Whi5-GFP nuclear index (green circles) of a representative elutriated daughter cell during growth in SC plus glucose. Completion of Whi5 export is indicated by a green arrowhead. Other parameters deduced from plotted data, volume at Start (Vs), volume growth rate in G1 (α) and time at Start (T1) are also indicated. (c) Volume at Start (Vs) versus growth rate in G1 (α) for asynchronous (black,n=100) or elutriated (red,n=78)WHI5-GFPdaughter cells growing in SC plus glucose. A linear regression line is plotted (r2>0.852). (d) Volume at Start (Vs) versus growth rate in G1 (α) for asynchronousWHI5-GFPdaughter cells growing in SC plus glucose (red,n=100,r2>0.852), galactose (green,n=100,r2>0.738), raffinose (orange,n=100,r2>0.683) or ethanol (blue,n=100,r2>0.733). A combined linear regression line is plotted (r2>0.919, seeSupplementary Table S1for details). (e,f) Volume at Start (Vs) versus time at Start (T1) for cells shown in panelscandd, respectively. (g,h) Time at Start (T1) versus volume growth rate in G1 (α) for cells shown in panelscandd, respectively. Figure 2: Volume at Start correlates with volume growth rate in G1 at a single-cell level. ( a ) Start can be defined as the event where Whi5 is exported from the nucleus [23] , [43] . Thus, time at Start ( T 1) was determined as the period where Whi5 was nuclear, whereas time to budding ( T 2) was the period from Whi5 exit from the nucleus to budding. Bar=2 μm. ( b ) Cell volume (black circles) and Whi5-GFP nuclear index (green circles) of a representative elutriated daughter cell during growth in SC plus glucose. Completion of Whi5 export is indicated by a green arrowhead. Other parameters deduced from plotted data, volume at Start ( V s), volume growth rate in G1 ( α ) and time at Start ( T 1) are also indicated. ( c ) Volume at Start ( V s) versus growth rate in G1 ( α ) for asynchronous (black, n =100) or elutriated (red, n =78) WHI5-GFP daughter cells growing in SC plus glucose. A linear regression line is plotted ( r 2 >0.852). ( d ) Volume at Start ( V s) versus growth rate in G1 ( α ) for asynchronous WHI5-GFP daughter cells growing in SC plus glucose (red, n =100, r 2 >0.852), galactose (green, n =100, r 2 >0.738), raffinose (orange, n =100, r 2 >0.683) or ethanol (blue, n =100, r 2 >0.733). A combined linear regression line is plotted ( r 2 >0.919, see Supplementary Table S1 for details). ( e , f ) Volume at Start ( V s) versus time at Start ( T 1) for cells shown in panels c and d , respectively. ( g , h ) Time at Start ( T 1) versus volume growth rate in G1 ( α ) for cells shown in panels c and d , respectively. Full size image Growth rate during G1 governs cell size variability at Start One approach to studying whether a cell cycle transition is controlled by a sizer is to test whether smaller cells gain more size before the transition [44] , and this can be effected using an αT-plot, where increase in volume (that is, αT, the product of volume growth rate and time) is plotted against initial volume [37] , [44] , [45] . If cell volume at Start ( V s) were a constant determined by external conditions, αT 1 should correlate negatively with the initial volume ( V i) with a slope of −1 ( Fig. 3a ). Although we observed a negative correlation between αT 1 and V i in asynchronously growing cells, the slope was significantly different from −1 and the coefficient of determination was only 0.114, with data points being notably more scattered at small initial volumes ( Fig. 3b ; Supplementary Table S4 ). Very similar patterns have been interpreted to be the result of molecular noise inherent to the Start network [37] . However, we show here ( Fig. 2c, d ) that volume at Start ( V s) can be expressed as a linear function of the individual volume growth rate ( α ) by V s=k. α + V 0 , where V 0 is the minimum volume that a cell would attain at Start when its growth rate approaches zero, and k is a constant inherent to the sizer mechanism or, more formally, the time that a cell born with volume V 0 would always spend in G1 independently of its growth rate. Once this function was incorporated into the equation for αT 1, our data produced a completely different outcome ( Fig. 3c ). First, the slope was −0.91, a value not significantly different from −1 ( Supplementary Table S5 ). Second, the coefficient of determination increased to 0.783, with an evident decrease in the scatter for small newborn cells. Despite the fact that V i and T 1 for elutriated cells could only be estimated, the results obtained were comparable to those obtained from asynchronously growing cells ( Fig. 3b, c ). More importantly, the same correlation was obtained with cells growing in different carbon sources ( Fig. 3d, e ), and a single regression line could be fitted independently of the carbon source used as nutrient. Thus, we conclude that variation in the individual growth rate and not inherent molecular noise is what causes the main variability in cell volume at Start. 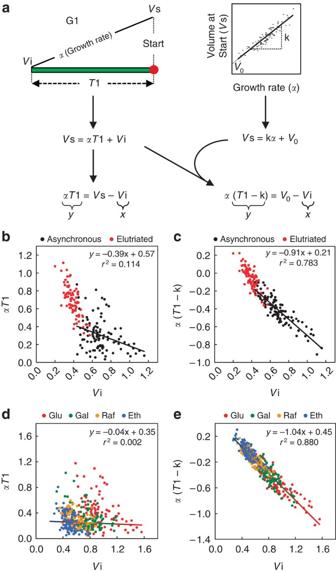Figure 3: Variability within the sizer mechanism is mainly due to individual differences in growth rate. (a) Assuming simple linear kinetics for volume growth in G1, volume at Start (Vs) can be expressed as a function of volume growth rate in G1 (α), time at Start (T1) and initial volume (Vi) byVs=αT1+Vi which, rearranging terms, yieldsαT1=Vs−Vi. If cell volume at Start (Vs) were constant,αT1 should correlate negatively with the initial volume (Vi) with slope of −1 (see text for details). However,Vs is a linear function of the individual volume growth rate (Vs=kα+V0) and, rearranging terms, it follows thatα(T1−k)=V0−Vi.V0is the minimum volume that a cell would attain at Start when its growth rate approaches zero and k is a constant inherent to the sizer mechanism or, more formally, the time that a cell born with volumeV0would always spend in G1 independently of its growth rate. (b,c) Cell volume (Vs), time at Start (T1) and volume growth rate in G1 (α) determined from individual asynchronous (black,n=100) or elutriated (red,n=78)WHI5-GFPdaughter cells growing in SC plus glucose were normalized with respect to the corresponding mean volume at Start, and used to generateαT1 (b) orα(T1−k) (c) versusVi plots. Regression lines obtained from asynchronous cells are plotted and corresponding slopes, intercepts and coefficients of determination (r2) are shown (seeSupplementary Tables S4-S5for details). (d,e) Cell volume (Vs), time at Start (T1) and volume growth rate in G1 (α) determined from individualWHI5-GFPdaughter cells asynchronously growing in SC plus glucose (red,n=100), galactose (green,n=100), raffinose (orange,n=100) or ethanol (blue,n=100) were made relative to the corresponding mean volume at Start, and used to generateαT1 (d) orα(T1−k) (e) versusVi plots. Regression lines are plotted and corresponding slopes, intercepts and coefficients of determination (r2) are shown (seeSupplementary Tables S4-S5for details). Figure 3: Variability within the sizer mechanism is mainly due to individual differences in growth rate. ( a ) Assuming simple linear kinetics for volume growth in G1, volume at Start ( V s) can be expressed as a function of volume growth rate in G1 ( α ), time at Start ( T 1) and initial volume ( V i) by V s= αT 1+ V i which, rearranging terms, yields αT 1= V s− V i. If cell volume at Start ( V s) were constant, αT 1 should correlate negatively with the initial volume ( V i) with slope of −1 (see text for details). However, V s is a linear function of the individual volume growth rate ( V s=k α + V 0 ) and, rearranging terms, it follows that α ( T 1−k)= V 0 − V i. V 0 is the minimum volume that a cell would attain at Start when its growth rate approaches zero and k is a constant inherent to the sizer mechanism or, more formally, the time that a cell born with volume V 0 would always spend in G1 independently of its growth rate. ( b , c ) Cell volume ( V s), time at Start ( T 1) and volume growth rate in G1 ( α ) determined from individual asynchronous (black, n =100) or elutriated (red, n =78) WHI5-GFP daughter cells growing in SC plus glucose were normalized with respect to the corresponding mean volume at Start, and used to generate αT 1 ( b ) or α ( T 1−k) ( c ) versus V i plots. Regression lines obtained from asynchronous cells are plotted and corresponding slopes, intercepts and coefficients of determination ( r 2 ) are shown (see Supplementary Tables S4-S5 for details). ( d , e ) Cell volume ( V s), time at Start ( T 1) and volume growth rate in G1 ( α ) determined from individual WHI5-GFP daughter cells asynchronously growing in SC plus glucose (red, n =100), galactose (green, n =100), raffinose (orange, n =100) or ethanol (blue, n =100) were made relative to the corresponding mean volume at Start, and used to generate αT 1 ( d ) or α ( T 1−k) ( e ) versus V i plots. Regression lines are plotted and corresponding slopes, intercepts and coefficients of determination ( r 2 ) are shown (see Supplementary Tables S4-S5 for details). Full size image Start network sets critical size as a function of growth rate Cells execute Start through a network of proteins ( Fig. 4a ) that ultimately activate the G1/S regulon. Accordingly, we tested whether these proteins have a direct impact on cell size regulation by growth rate ( Fig. 4 , Supplementary Tables S1-S5 ). First, we analysed the role of two well-characterized inhibitors of Start: Whi3 and Whi5. Whi3 binds the CLN3 mRNA and contributes to retain the Cdc28–Cln3 complex in the cytoplasm in G1 cells [31] , [32] . On the other hand, Whi5 [22] , [23] binds G1/S transcription factors [14] to inhibit their activity in the nucleus during G1. Thus, we analysed cells deficient for Whi3 ( Fig. 4b ) or expressing whi5N ( Fig. 4c ), which produces an N-terminal fragment of Whi5 unable to inhibit the G1/S transition but still subject to cell-cycle-regulated export [46] . A priori, we expected that smaller cells at Start could be obtained by decreasing either k, the slope inherent to the sizer mechanism that defines the linear growth rate dependency, or V 0 , the minimal volume at Start for a cell with a growth rate approaching zero. We found that size at Start for both whi3 and whi5N cells was still dependent on the individual volume growth rate, but with a much smaller slope k compared with wild-type cells, indicating that both inhibitors participate in the sizer mechanism by linking cell size at Start to volume growth rate in G1. The small cell size phenotype is particularly important at high growth rates, which indicates that both negative regulators are needed in the mechanisms by which growth inhibits Start [4] , [47] . 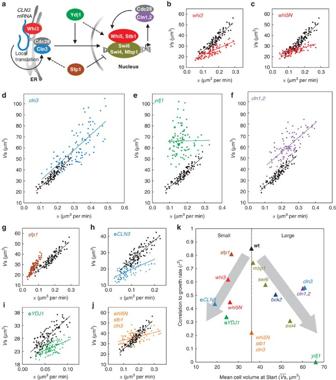Figure 4: The Start network sets cell size as a function of the individual growth rate in G1. (a) Scheme of the Start network with components and interactions. Briefly, the Cdk–cyclin complex formed by Cln316,17,18,19,20and Cdc2821phosphorylates the transcriptional repressor Whi522,23and activates SBF (Swi6/Swi4) and MBF (Swi6/Mbp1) transcription factors14to induce the G1/S regulon15and trigger cell cycle entry. Whi3 and Ydj1 act as negative and positive regulators, respectively, of release of cyclin Cln3 from the ER31,32,33to allow its accumulation in the nucleus. Perhaps, indirectly, Ydj1 could also be required for proper SBF and MBF function (dashed arrow). Cln1 and Cln2 cyclins generate a positive feedback loop essential for coherent and robust SBF and MBF activation25,26,27, and Stb1 is a transcriptional modulator that contributes to inhibit SBF- and MBF-dependent transcription during G148. Sfp1 acts as a negative regulator of Start (continuous arrow) and, as it is a transcription activator in ribosome biogenesis, Sfp1 would also upregulate Cln3 levels (dashed arrow) as a result of increased translation4. (b–j) Volume at Start versus volume growth rate in G1 for wild-type (black),whi3(b, red),whi5N(c, dark red),cln3(d, blue),ydj1(e, green),cln1,2(f, purple),sfp1(g, brown), oCLN3(h, blue), oYDJ1(i, green) andcln3 whi5N stb1(j, orange) daughter cells (n=100). All strains expressedWHI5-GFPorwhi5N-GFPfusion proteins and were analysed in SC plus glucose. (k) Correlation (r2) between individual growth rate and volume at Start as a function of mean cell volume at Start for the indicated strains. Figure 4: The Start network sets cell size as a function of the individual growth rate in G1. ( a ) Scheme of the Start network with components and interactions. Briefly, the Cdk–cyclin complex formed by Cln3 [16] , [17] , [18] , [19] , [20] and Cdc28 [21] phosphorylates the transcriptional repressor Whi5 [22] , [23] and activates SBF (Swi6/Swi4) and MBF (Swi6/Mbp1) transcription factors [14] to induce the G1/S regulon [15] and trigger cell cycle entry. Whi3 and Ydj1 act as negative and positive regulators, respectively, of release of cyclin Cln3 from the ER [31] , [32] , [33] to allow its accumulation in the nucleus. Perhaps, indirectly, Ydj1 could also be required for proper SBF and MBF function (dashed arrow). Cln1 and Cln2 cyclins generate a positive feedback loop essential for coherent and robust SBF and MBF activation [25] , [26] , [27] , and Stb1 is a transcriptional modulator that contributes to inhibit SBF- and MBF-dependent transcription during G1 [48] . Sfp1 acts as a negative regulator of Start (continuous arrow) and, as it is a transcription activator in ribosome biogenesis, Sfp1 would also upregulate Cln3 levels (dashed arrow) as a result of increased translation [4] . ( b–j ) Volume at Start versus volume growth rate in G1 for wild-type (black), whi3 ( b , red), whi5N ( c , dark red), cln3 ( d , blue), ydj1 ( e , green), cln1,2 ( f , purple), sfp1 ( g , brown), o CLN3 ( h , blue), o YDJ1 ( i , green) and cln3 whi5N stb1 ( j , orange) daughter cells ( n =100). All strains expressed WHI5-GFP or whi5N-GFP fusion proteins and were analysed in SC plus glucose. ( k ) Correlation ( r 2 ) between individual growth rate and volume at Start as a function of mean cell volume at Start for the indicated strains. Full size image We next analysed the role of Cln3, the most upstream G1 cyclin that activates Start [16] , [17] , [18] , [19] , [20] . We observed a clear dependence of cell size at Start on growth rate in Cln3-deficient cells ( Fig. 4d ), and similar results were obtained with cells lacking both Cln1 and Cln2 ( Fig. 4f ), the two G1 cyclins that contribute to Start in a positive feedback loop [25] , [26] , [27] . Thus, rather than being mediators, individual G1 cyclins would be target effectors of the sizing mechanism. However, Cln3- and Cln1,2-deficient cells showed a lower correlation between volume at Start and growth rate, indicating that their cooperative presence is important to achieve a robust growth-rate-dependent size control. Cells deficient for Ydj1, the J-chaperone that releases the Cdc28–Cln3 complex from the ER to trigger Start [33] , were much larger than wild-type as expected but, more important, there was no correlation between cell volume at Start and volume growth rate in G1 ( Fig. 4e ). This result indicates that this chaperone is essential to determine cell size at Start as a function of growth rate. Ribosome biogenesis activators Sfp1 and Sch9 also act as important negative regulators of Start [34] , [47] . As described, we found that Sfp1-deficient cells were smaller than wild-type [34] , but cell volume at Start still showed a very strong correlation with growth rate in G1 ( Fig. 4g ), suggesting that ribosome biogenesis regulates size as an upstream determinant of growth rate. In addition, as the correlation function was steeper in sfp1 than wild-type cells, Sfp1 could also have a positive role at Start, possibly by increasing translation rates and Cln3 levels [4] . Cln3 and Ydj1 are both rate limiting for cell cycle entry [19] , [33] and, as expected, their overexpression decreased the average cell volume at Start ( Supplementary Table S6 ). Both the slope of the correlation function and the coefficient of determination were also smaller in o CLN3 ( Fig. 4h ) and o YDJ1 ( Fig. 4i ) cells, indicating that unusually high levels of Cln3 or Ydj1 produce a small cell size at Start because they weaken its dependence on growth rate in a similar manner to the lack of negative regulators Whi3 or Whi5. Cells simultaneously lacking activating (Cln3) and inhibiting (Whi5, Stb1) components of the Start network display a budding size very similar to wild-type cells [48] . Accordingly, when we analysed cln3 whi5N stb1 cells by time-lapse microscopy, we found that average cell volume at Start was very similar to wild-type cells ( Supplementary Table S6 ). However, correlation of individual cell volume at Start to growth rate in G1 was almost lost ( Fig. 4j ). In summary, although deletion or overexpression of components of the Start network causes small or large cell phenotypes consistent with their positive or negative role, all these genetic alterations loose the strong dependency of the critical size on growth rate ( Fig. 4k ). Thus, a key role of the Start network in regulating cell size is by setting it as a function of growth rate for each individual cell. Role of a growth-rate-dependent sizer To test whether a growth-rate-dependent sizer is able to ensure size homeostasis at a population level, we used our experimental data to model growth in volume during the yeast cell cycle ( Fig. 5a ; a detailed description can be found in Supplementary Methods ). We assumed that volume at Start is a stochastic variable that depends on growth rate, and we used two different approaches for modelling, a germline ( Fig. 5b and Supplementary Data 1 ) and a pedigree algorithm ( Fig. 6a and Supplementary Software 1 ). Validating their design, both modelling approaches predicted the observed independence of time to Start ( T 1) on growth rate ( α ), and produced αT -plots very similar to the experimental data ( Fig. 5c,d and Supplementary Fig. S6 ). Predicted values for all dependent variables, that is, G1 length and volumes at the beginning of G1, Start, budding and division, were not significantly different from experimental data ( Fig. 5e ). Starting from a single cell, the pedigree approach generated a stable variability in daughter cell volume at Start in less than 10 generations ( Fig. 6b ) and predicted that mother cells should increase their volume in each generation ( Fig. 6c ) as experimentally observed [13] , [49] . Moreover, the pedigree analysis produced steady-state cell size distributions very similar to the experimental data obtained in different nutritional conditions ( Fig. 6d ). Germline modelling predicted a stable pattern of fluctuations in daughter cell volume at Start over 1,000 generations ( Fig. 7c ). As expected, much larger fluctuations were predicted by our model if volume growth rate in a cell cycle phase was made to depend on the initial volume at that phase ( Supplementary Fig. S7 ). However, we found that growth rates in G1 ( α ) and S–G2–M ( β ) do not correlate with the respective initial volumes ( Supplementary Fig. S7 ). Overall, both modelling approaches indicate that a single growth-rate-dependent size control within the cell cycle is sufficient to maintain cell size homeostasis. 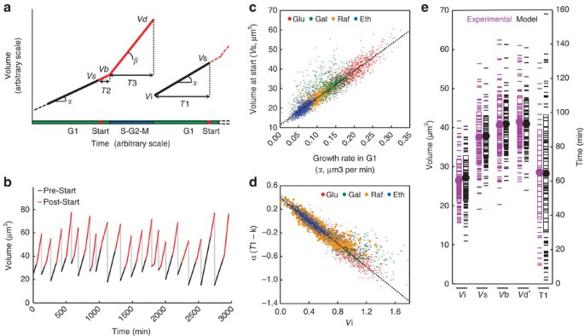Figure 5: The germline method as a model of volume growth during the budding yeast cycle. (a) Scheme with variables and relationships used to design a stepwise model of volume growth during the cell cycle of budding yeast. Independent (experimental, bold symbols) and dependent (produced by the model) variables are specified. Equations for each step are described inSupplementary Methods. (b) The germline method was used to simulate volume growth of daughter cells for 20 consecutive cycles. Pre-Start (black lines) and post-Start (red lines) periods are indicated. (c) Volume at Start (Vs) versus growth rate in G1 (α) for daughter cells growing in SC plus glucose (red,n=1,000), galactose (green,n=1,000), raffinose (orange,n=1,000) or ethanol (blue,n=1,000) simulated by the germline method. The regression line (dotted line) obtained from experimental data inFigure 2dis also shown. (d) Cell volume (Vs), time at Start (T1) and volume growth rate in G1 (α) determined from daughter cells as incwere made relative to the corresponding mean volume at Start, and used to generate aα(T1−k) versusVi plot. The regression line (dotted line) obtained from experimental data inFigure 3eis also shown. (e) Volumes at the beginning of G1 (Vi), Start (Vs), budding (Vb) and division (Vd', only mother compartment), and time at Start (T1) for daughter cells growing in SC plus glucose from experimental data (purple,n=100) or simulated by the germline method (black,n=100). Mean (circles) and s.d. intervals (boxes) are shown. Figure 5: The germline method as a model of volume growth during the budding yeast cycle. ( a ) Scheme with variables and relationships used to design a stepwise model of volume growth during the cell cycle of budding yeast. Independent (experimental, bold symbols) and dependent (produced by the model) variables are specified. Equations for each step are described in Supplementary Methods . ( b ) The germline method was used to simulate volume growth of daughter cells for 20 consecutive cycles. Pre-Start (black lines) and post-Start (red lines) periods are indicated. ( c ) Volume at Start ( V s) versus growth rate in G1 ( α ) for daughter cells growing in SC plus glucose (red, n =1,000), galactose (green, n =1,000), raffinose (orange, n =1,000) or ethanol (blue, n =1,000) simulated by the germline method. The regression line (dotted line) obtained from experimental data in Figure 2d is also shown. ( d ) Cell volume ( V s), time at Start ( T 1) and volume growth rate in G1 ( α ) determined from daughter cells as in c were made relative to the corresponding mean volume at Start, and used to generate a α ( T 1−k) versus V i plot. The regression line (dotted line) obtained from experimental data in Figure 3e is also shown. ( e ) Volumes at the beginning of G1 ( V i), Start ( V s), budding ( V b) and division ( V d', only mother compartment), and time at Start ( T 1) for daughter cells growing in SC plus glucose from experimental data (purple, n =100) or simulated by the germline method (black, n =100). Mean (circles) and s.d. intervals (boxes) are shown. 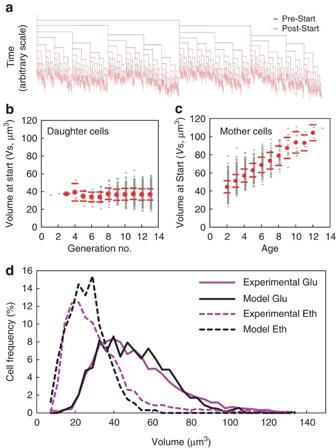Figure 6: Population predictions of cell volume using the pedigree method. (a) The pedigree method was used to simulate the whole progeny of a single cell for 10 generations and the time extent of pre-Start (black lines) and post-Start (red lines) periods is represented. (b) Volume at Start (Vs) for daughter cells in 13 consecutive generations as predicted by the pedigree method. Individual (grey small symbols), mean (red circles) and s.d. interval values (red bars) are shown. (c) Volume at Start (Vs) for mother cells as a function of age by the pedigree method. Individual (grey small symbols), mean (red circles) and s.d. interval values (red bars) are shown. (d) Volume distributions of cells growing asynchronously under steady-state conditions in SC plus glucose (continuous lines) or ethanol (broken lines) were obtained with a Coulter Counter (purple lines,n>10000) or were simulated by the pedigree method (black lines). Full size image Figure 6: Population predictions of cell volume using the pedigree method. ( a ) The pedigree method was used to simulate the whole progeny of a single cell for 10 generations and the time extent of pre-Start (black lines) and post-Start (red lines) periods is represented. ( b ) Volume at Start ( V s) for daughter cells in 13 consecutive generations as predicted by the pedigree method. Individual (grey small symbols), mean (red circles) and s.d. interval values (red bars) are shown. ( c ) Volume at Start ( V s) for mother cells as a function of age by the pedigree method. Individual (grey small symbols), mean (red circles) and s.d. interval values (red bars) are shown. ( d ) Volume distributions of cells growing asynchronously under steady-state conditions in SC plus glucose (continuous lines) or ethanol (broken lines) were obtained with a Coulter Counter (purple lines, n >10000) or were simulated by the pedigree method (black lines). 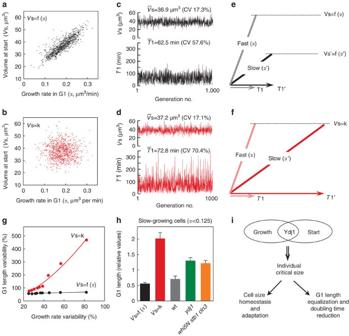Figure 7: The growth-rate-dependent sizer achieves size homeostasis and prevents unwanted large variations of G1 length. (a,b) Volume at Start (Vs) versus volume growth rate in G1 (α) of daughter cells (n=1,000) growing in SC plus glucose predicted by the germline method assuming that volume at Start is a stochastic variable that depends on growth rate (a;Vs=f[α]) or not (b;Vs=k). (c,d) Volume at Start (Vs) and time at Start (T1) fluctuations over 1,000 generations as predicted by the germline method are shown assuming that volume at Start depends on growth rate (c;Vs=f(α)) or not (d;Vs=k). Average data and coefficients of variation (in parenthesis) are also shown. (e,f) Slow growing cells display much shorter G1 periods comparing growth-rate-dependent (e;Vs=f(α)) to independent (f;Vs=k) sizer mechanisms. In other words, slow-growing cells must grow for a longer time if the critical size is not reduced as a function of growth rate. (g) G1 length variability was predicted as a function of growth rate variability by the germline method assuming that volume at Start depends on growth rate (Vs=f(α), black circles) or not (Vs=k, red circles). Values are plotted as coefficients of variation (%). (h) Average G1 length of slow growing cells (α<0.125 μm3per min) predicted by the model assuming that volume at Start depends (Vs=f(α)) or not (Vs=k) on growth rate. Experimental data for wild-type,ydj1andwhi5N stb1 cln3cells are also shown. G1 length values were made relative to the average of all cells for each simulation condition or strain, and mean values and confidence limits for the mean (significance level of 0.05) are plotted. (i) Our data reveal the existence of a deterministic size control that sets cell size as a function of growth rate at a single cell level. Although robustness of the mechanism requires all Start network components, we have found that Ydj1 has the most essential role in the growth-dependent sizer, which not only provides with size homeostasis and adaptation, but also allows for G1 length equalization to reduce the generation time at a population level. Full size image Figure 7: The growth-rate-dependent sizer achieves size homeostasis and prevents unwanted large variations of G1 length. ( a , b ) Volume at Start ( V s) versus volume growth rate in G1 ( α ) of daughter cells ( n =1,000) growing in SC plus glucose predicted by the germline method assuming that volume at Start is a stochastic variable that depends on growth rate ( a ; V s=f[ α ]) or not ( b ; V s=k). ( c , d ) Volume at Start ( V s) and time at Start ( T 1) fluctuations over 1,000 generations as predicted by the germline method are shown assuming that volume at Start depends on growth rate ( c ; V s=f( α )) or not ( d ; V s=k). Average data and coefficients of variation (in parenthesis) are also shown. ( e , f ) Slow growing cells display much shorter G1 periods comparing growth-rate-dependent ( e ; V s=f( α )) to independent ( f ; V s=k) sizer mechanisms. In other words, slow-growing cells must grow for a longer time if the critical size is not reduced as a function of growth rate. ( g ) G1 length variability was predicted as a function of growth rate variability by the germline method assuming that volume at Start depends on growth rate ( V s=f( α ), black circles) or not ( V s=k, red circles). Values are plotted as coefficients of variation (%). ( h ) Average G1 length of slow growing cells ( α <0.125 μm 3 per min) predicted by the model assuming that volume at Start depends ( V s=f( α )) or not ( V s=k) on growth rate. Experimental data for wild-type, ydj1 and whi5N stb1 cln3 cells are also shown. G1 length values were made relative to the average of all cells for each simulation condition or strain, and mean values and confidence limits for the mean (significance level of 0.05) are plotted. ( i ) Our data reveal the existence of a deterministic size control that sets cell size as a function of growth rate at a single cell level. Although robustness of the mechanism requires all Start network components, we have found that Ydj1 has the most essential role in the growth-dependent sizer, which not only provides with size homeostasis and adaptation, but also allows for G1 length equalization to reduce the generation time at a population level. Full size image Finally, we took advantage of the germline modelling approach to compare the growth-rate-dependent sizer with the steady sizer generally assumed up to now ( Fig. 7a,b ). Notably, G1 length fluctuations were much smaller for growth-rate-dependent ( Fig. 7c ) versus constant ( Fig. 7d ) sizer mechanisms. The predicted difference is so important that the average generation time for the population would be approximately 15% longer if critical size did not depend on growth rate. This effect is mainly due to slow-growing cells, because they have to grow for a longer time when the critical size is not reduced as a function of growth rate ( Fig. 7e, f ). Thus, G1 length variability is insensitive to growth rate variation only for the growth-rate-dependent sizer ( Fig. 7g ). As they showed no significant correlation between volume at Start and growth rate, ydj1 and whi5N stb1 cln3 cells would behave as if they were subject to a constant sizer mechanism. Indeed, slow-growing cells of both mutant strains displayed a clear increase in G1 length compared with wild-type cells with same growth rate ( Fig. 7h ). Our methodological approach to accurately determine the optical cell boundary has allowed us to observe a clearly discontinuous pattern of growth in volume during the cell cycle of budding yeast. Growth rate in volume was rather constant during G1 and it only showed a slight decrease immediately before budding. Notably, average volume growth rate in G2–M increased 2.3-fold compared with G1 phase. Mitchison [41] had shown the existence of an RCP for growth in volume shortly after budding. On the other hand, although cell volumes were estimated from protein concentration, a recent report also has given support to this notion [42] . As protein synthesis seems to increase exponentially during the cell cycle [37] , [42] , [50] , [51] , a discontinuous pattern of growth in volume should cause changes in cell density over the cell cycle, consistent with the fact that yeast cells reach a maximum density shortly after budding [52] , [53] . All these observations point to a discontinuous mode of volume growth during the cell cycle of budding yeast, a property that has been well established in the fission yeast Schizosaccharomyces pombe [44] , [45] , [54] and may also apply to mammalian cells [55] . Finally, from an opposite but complementary point of view, it is clear that cell growth is in turn governed by cell cycle progression [56] ; so, in addition to gene-dosage effects as a result of DNA replication, shifting growth from apical to isotropic modes in G2 could give raise to the observed RCP. It is generally accepted that budding yeast cells must reach a critical size before entering the cell cycle [12] , [13] . Nevertheless, individual cells offer a large variability in their size at Start under constant external and nutritional conditions [36] , [37] , and this fact has seriously challenged the existence of a deterministic mechanism setting the critical size in a dedicated manner. We have found that yeast cells set their size at Start as a robust function of the individual growth rate, the observed population variability in size at Start being a consequence of the intrinsic variation of growth rate in volume among cells. Our findings clearly support a deterministic mode of cell size control and rule out the notion of a universal critical size that, once defined by external conditions, had to be satisfied by all cells in the population to enter the cell cycle. Concerning the variability in volume growth rate, similar variations in different biosynthetic processes have already been reported in yeast [38] , [39] , [40] . However, we have found no (or very weak) correlations between volume growth rate and either ribosomal protein levels, GFP synthesis rates or ER contents (F.F., N.C. and M.A, unpublished results). Growth in volume is a very complex process, with many different factors likely suffering from some stochastic behaviour, which altogether could cause a large variability in the overall rate. The dependency of cell size at Start on growth rate in G1 was extremely dependent on the proteins that control entry into the cell cycle and thus define the Start network. Small cells lacking negative regulators (Whi3, Whi5) or overexpressing positive effectors (Cln3, Ydj1) still showed a growth-rate-dependent volume at Start, but with lower coefficients of correlation compared with wild-type cells. Loss of G1 cyclins Cln3 or Cln1,2, or G1/S transcription factors, which produce a large-cell phenotype, also caused a decrease in the correlation between volume at Start and growth rate in G1. Moreover, cells simultaneously lacking activating (Cln3) and inhibiting (Whi5, Stb1) components of the Start network displayed a much weaker correlation of cell volume at Start to growth rate in G1, indicating that the Start network is deeply involved in the growth-rate-dependent sizer mechanism. Notably, loss of Ydj1 caused the most severe effects in the dependency of the critical size on growth rate. As Ydj1 is also involved in cell wall growth processes, such as protein translocation at the ER [35] , our data suggest that the key molecular device operating this correlation is at the interface between the cell cycle and cell growth machineries. In this regard, ribosome biogenesis activators Sfp1 and Sch9 also act as important negative regulators of Start [47] . However, we found that Sfp1-deficient cells still showed a very strong correlation between cell size at Start and growth rate in G1, which suggests that ribosome biogenesis would determine the critical size through its immediate effects on growth rate. On the basis of a mathematical model of volume growth during the yeast cell cycle, we have shown that a growth-rate-dependent sizer is able to provide size homeostasis only if growth rate is made independent of the initial cell volume. Notably, we have found that growth rates in G1 and G2–M do not depend on the respective initial volumes, which confirms similar results obtained from α -factor-arrested cells in G1 ( Supplementary Fig. S2b–d in ref. 39 ). An intrinsic control that sets the critical size as a function of growth rate also provides a broad solution for adaptation, thus making unnecessary the existence of a plethora of sensing mechanisms transmitting different external cues to the cell cycle machinery. Our experimental data suggest that, in addition to provide with homeostasis and adaptation, a growth-rate-dependent sizer would reduce noise in G1 length, which would in turn prevent loss of slow-growing cells and shorten the generation time at the population level ( Fig. 7i ). As slow-growing cells show a longer lifespan, these effects would provide the population with a significant evolutionary advantage. Although robustness of the mechanism requires all Start network components, we have found that Ydj1 has the most essential role in dictating the critical size as a function of growth rate. We have proposed that high volume growth rates should require higher levels of chaperones at ribosome biogenesis, protein synthesis and protein translocation, thus decreasing available chaperone levels for other processes, such as Cln3 release from the ER [29] . As a consequence, a fast-growing cell would delay cell cycle entry until it has grown large enough and has accumulated sufficient chaperone levels to trigger Start. Indeed, our work demonstrates that budding yeast cells set their critical size at a single-cell level as a function of growth rate in volume and supports a model whereby competition for molecular chaperones could subordinate proliferation to growth and help cells to attain an individually tailored size. Strain constructions BY4741 WHI5::GFP [57] (supplied by Invitrogen) and CML128 (a S288C derivative [58] ) were used as wild-type strains of Saccharomyces cerevisiae . Standard PCR-based gene-replacement methods were used to obtain the indicated deletions, C-terminal translational fusions to GFP and mCherry, or transcriptional fusions to the GAL1 promoter at the respective chromosomal loci. To analyse Whi5-deficient cells, we used a GFP fusion of the N-terminal fragment of Whi5 ( whi5N ) unable to inhibit the G1/S transition but still subject to cell-cycle-regulated export [46] . Growth conditions Cells were grown under exponential conditions for at least 14 h in synthetic complete (SC) medium [59] with either 2% glucose, 2% galactose, 2% raffinose or 3% ethanol at 30 °C before microscopy. CLN3 and YDJ1 overexpression was attained adding 2% galactose to cells that contained transcriptional fusions to the GAL1 promoter at the respective chromosomal loci. CLN3 overexpression ( oCLN3 ) was evaluated in asynchronous daughter cells growing in SC plus galactose. YDJ1 overexpression ( oYDJ1 ) was assessed in daughter cells elutriated 3 h after adding galactose to a culture grown in raffinose. As they contained a MET3p-CLN2 construct to avoid accumulation of aberrantly shaped cells, cln1,2 cells were grown in SC medium without methionine, which was added immediately before the time-lapse experiment [27] . Newly born cells were obtained by elutriation [19] . Coverslips (25 mm) were precoated at a small central area with 0.1 ml 0.1mg ml −1 concanavalin A type V (Sigma-Aldrich) in water for 60 min in a humid chamber, washed twice with water and kept at 4 °C in water for up to 24 h before use [39] . Cells (0.1 ml, optical density at 600 nm (OD 600 )=0.5) were added to the coverslip and left at room temperature for 2 min to obtain 20–40 bound cells per field. After two washes with 0.1 ml SC medium to remove unbound cells, the coverslip was assembled in a prewarmed RC-43C chamber (Warner Instruments, www.warneronline.com ) with ca. 0.3 ml SC medium, such that concentration of bound cells within the chamber would correspond to an OD 600 lower than 0.1. When elutriated cells were analysed, they were first suspended in SC medium at OD 600 =2 and bound to the centre of a concanavalin A-coated round 25-mm coverslip. Temperature at the centre of the chamber was maintained at 30±1 °C with the help of a DH-40i micro-incubator system and a Single Channel Heater Controller TC-324B (Warner Instruments). Time-lapse microscopy Cells were imaged by time-lapse microscopy under a fully motorized Axio Observer Z1 inverted microscope (Zeiss) equipped with a Plan-Apochromat ×100/1.40 objective, differential interference contrast (DIC) optics, an XY-motorized stage, a 100 W mercury lamp controlled by a FluoArc unit (Zeiss), adequate filters for GFP and mCherry detection, and an AxioCam MRm camera (Zeiss). Typically, 14 fields were automatically and repeatedly analysed every 3 min for 180 min using AxioVision 4.1 software (Zeiss) to obtain DIC, bright-field and fluorescence images. Autofocus was applied to the DIC image with a 50% threshold, and an offset of 1 μm was required to correct for an invariable deviation and obtain a precise focus of the cells before imaging. An additional offset of 1 μm was applied before taking the bright-field image to obtain the highest contrast at the cell boundary. To minimize irradiation of the cells, which were exposed for 1 s to obtain fluorescence images, illumination from the mercury lamp was reduced to 5% with the help of an appropriate neutral filter and the FluoArc unit. A diaphragm slider was used to limit illumination to the imaged field. A small percentage of cells (less than 2%) failed to grow and were not analysed further. Under these conditions, the average growth rate in cell volume was comparable to that obtained with a Coulter Counter from a batch culture ( Supplementary Fig. S1 ). In addition, average growth rates from fields imaged or not for fluorescence were not significantly different ( Supplementary Fig. S1 ). Image analysis and cell measurements We obtained cell dimensions from bright-field images (see ref. 60 for a discussion on the use of fluorescence or bright-field images for identifying cell boundaries). Specific procedures in Visual Basic using object libraries supplied by AxioVision (Zeiss) software were written to detect cell boundaries as pixels markedly darker compared with both the surrounding background and the cell interior. The algorithm first obtains a densitometric profile along a radial axis from a seed point within the cell (initially provided by the user) to find two consecutive maximum and minimum pixel values produced around the cell boundary, which is arbitrarily established at an intermediate pixel having their arithmetic grayscale mean as value ( Fig. 1b ; Supplementary Movie 2 ). Then, cell boundary pixels are iteratively defined by full rotation of the radial axis and a preliminary ellipse object is fitted. Outliers are first eliminated by their distance to the centre of the ellipse when it is larger than a fixed value. Second, additional outliers are eliminated when their distance to neighbour boundary pixels is larger than a fixed value. Once outliers have been removed, missing boundary pixels are estimated by fitting ellipsoidal segments. This process was essential to analyse daughter cells before cell separation. A final ellipse is then fitted to the obtained boundary pixel array, and major and minor axes are used to calculate the cell volume assuming a prolate as shape. The cell was followed through consecutive time-lapse images by using the centre of the ellipse as seed point to obtain radial profiles in the following time-point image. Volume distributions generated from time-lapse microscopy data were similar to those obtained with the Coulter Counter in batch cultures ( Supplementary Fig. S1 ). These procedures have been rewritten in Java as BudJ, an ImageJ plugin that can be obtained from www.ibmb.csic.es\home\maldea or, see Supplementary Software 2 . Quantification of Whi5 nuclear localization To avoid colocalization with a compatible fluorescent nuclear marker, which would necessarily increase light damage during growth, Whi5 localization in the nucleus was assessed as a relative index inversely proportional to the mean distance of the brightest pixels to their gravity centre ( Supplementary Fig. S4 ). Once cell boundaries are determined as described above, brightest pixels within the cell are first selected having a grey value larger than the mean plus two s.d. Next, the mean distance to their gravity centre is calculated and made relative to 8r/15, the theoretical mean distance to the centre from random points in a sphere projected to a circle with radius r . The nuclear index thus obtained when Whi5 has been already exported to the cytoplasm was very close to one ( Fig. 2b ). In addition, this approach produced results that correlated well with those obtained by colocalization with Htb2-mCherry as a nuclear marker ( Supplementary Fig. S4 ). Briefly, the Htb2-mCherry image was thresholded to obtain a binary mask and delimit nuclear and cytoplasmic regions within each cell identified in the bright-field image as described above. Next, colocalization was calculated as the mean brightness of pixels within the nuclear region made relative to that of pixels within the cytoplasmic compartment. Determination of cell parameters Growth rates in volume during G1 phase ( α ) were obtained by linear regression of volume data during this time period. Occasionally, a change in rate was clearly observed within G1, and in this case, individual growth rate in volume was obtained by linear regression of volume data during the 60 min before Whi5 nuclear export. Instantaneous growth rates as a function of time during G1 were estimated from data ±6 min around every time point. In asynchronous cultures, T 1 was the time period from Whi5 import to Whi5 export (Start), and T 2 was the time period from Start to budding. Once nuclear index values were smoothed by a sliding mean over three consecutive points, we defined Whi5 nuclear entry as the first time point with a nuclear index significantly different from 1, and Whi5 nuclear export as the first time point with a nuclear index not significantly different from 1. In elutriation experiments, we collected less than 0.2% of the cells loaded in the rotor, being the smallest cells among all newly born cells in the asynchronous culture. We could only approximate T 1 in elutriated cells as the period from time 0 (when we placed the newborn cells in the chamber with prewarmed medium) to Whi5 nuclear export. Thus, true V i and T 1 values for elutriated cells are expected to be slightly smaller and longer, respectively, than those measured. Initial cell volumes ( V i) and volumes at Start ( V s) and budding ( V b) were obtained directly from raw data of the corresponding time points. T3 was the time at division and was approximated as the time from budding to Whi5 import to the nucleus. Similarly, volume at division ( V d) was also obtained at Whi5 import. Although growth rates for the G2–M period were estimated by linear regression of volume data from 30 to 60 min after budding, growth rates for the S-G2–M period ( β ) were obtained as ( V d– V b)/T3. Finally, a few cells (less than 5% of all cells analysed) did not trigger Start during the course of the experiment or displayed growth rate differences to the average larger than two s.d. and were discarded as outliers. How to cite this article: Ferrezuelo, F. et al . The critical size is set at a single-cell level by growth rate to attain homeostasis and adaptation. Nat. Commun. 3:1012 doi: 10.1038/ncomms2015 (2012).